Electrifying photonic metamaterials for tunable nonlinear optics Metamaterials have not only enabled unprecedented flexibility in producing unconventional optical properties that are not found in nature, they have also provided exciting potential to create customized nonlinear media with high-order properties correlated to linear behaviour. Two particularly compelling directions are active metamaterials, whose optical properties can be purposely tailored by external stimuli in a reversible manner, and nonlinear metamaterials, which enable intensity-dependent frequency conversion of light waves. Here, by exploring the interaction of these two directions, we leverage the electrical and optical functions simultaneously supported in nanostructured metals and demonstrate electrically controlled nonlinear optical processes from a metamaterial. Both second harmonic generation and optical rectification, enhanced by the resonance behaviour in the metamaterial absorber, are modulated externally with applied voltage signals. Our results reveal an opportunity to exploit optical metamaterials as self-contained, dynamic electro-optic systems with intrinsically embedded electrical functions and optical nonlinearities. Optical metamaterials afford exotic light manipulation through artificial structuring and arranging of nanosized metal-dielectric subunits [1] , [2] , [3] , [4] , [5] . As the study of metamaterials evolves beyond the conventional, linear regime, an ever-growing emphasis is being placed on functionalizing these novel optical media into meta-devices for signal processing, light switching and sensing applications [6] , [7] , [8] , [9] . Although the linear responses of optical metamaterials have been extensively studied, the nonlinear phenomena in metamaterials, which usually form the basis for the dynamic response and active control of these novel media [10] , [11] , [12] , [13] , [14] , are comparably underdeveloped. The capability to design custom nonlinear materials, which is made possible through metamaterials, is bound to open entirely new vistas for nonlinear light–matter interactions. In optical metamaterials, nanostructured metals are cherished because of their unique plasmonic responses. Often neglected in this context is the fact that metals are electrically and thermally conductive, therefore enabling a range of secondary functions, including voltage offset, carrier injection and heat sinking. Consequently, optical metamaterials can be viewed as a self-contained electrooptic system with intrinsically embedded electrical functions. Electrically controlled optical functionalities enable a wide range of intriguing phenomena in both the linear and the nonlinear regimes. Taking second-order wave mixing as an example, nonlinear interactions such as second-harmonic generation (SHG, ω + ω →2 ω ) and optical rectification (OR, ω − ω →0) rely on the second-order nonlinear susceptibility, which is typically limited to crystals lacking a centre of inversion symmetry. In sharp contrast to conventional SHG and OR processes, application of a bias voltage across an optical medium can facilitate electric-field-induced second-harmonic (EFISH) generation and OR (EFIOR), which are third-order nonlinear effects enabled by an externally applied static or low-frequency field ( ω + ω +0→2 ω for EFISH and ω − ω +0→0 for EFIOR). As a result, these two electrically induced nonlinear phenomena are not limited to non-centrosymmetric materials with a non-zero χ (2) . Instead, the generation of EFISH and EFIOR signals is possible in all materials, because of the ubiquity of the third-order nonlinear susceptibility χ (3) . The EFISH effect was discovered in 1962, just 1 year after the first demonstration of SHG [15] , [16] and has been used in electrooptic applications such as the characterization of organic nonlinear materials and the ultrafast detection of electrical signals in semiconductors. Very recently, EFISH was brought to nanophotonic systems for the first time and was generated inside a polymer-filled plasmonic nanoslit [17] . Although both SHG and OR were discovered during the early days of nonlinear optics in the 1960s [18] , OR received very limited attention for decades until being revived as a major scheme for generating terahertz radiation [19] , [20] , [21] . The EFIOR was first demonstrated in 1977 where kilovolts of potential difference (corresponding to an electric field magnitude of ~1 V μm −1 ) were applied across a centrosymmetric nonlinear medium sandwiched between two electrodes [22] . In this work, we leverage the resonance-enhanced light-concentrating abilities of a metamaterial absorber and its electrical functions supported by the same nanostructured metal to experimentally demonstrate electrically induced and voltage-controlled nonlinear processes from an optical metamaterial. The second-harmonic and OR signals from the meta-device stem from an effective second-order response produced in the amorphous dielectric layer of the metamaterial by the interplay between the third-order nonlinear susceptibility and the applied control field ( ). Both the SHG and OR, enhanced by the resonance behaviour in the metamaterial, are modulated by applied voltage signals in a linear manner. This work represents an entirely new category of active metamaterials where nonlinear optical interactions can be purposely controlled by electrical signals. A metamaterial for electrically controlled nonlinear effect In this work, a dual-layered nanometallic absorber is employed to demonstrate voltage-controlled nonlinear optical processes. This type of metamaterial-based perfect absorber can be designed to capture all the energy of the incident light within a prescribed frequency range [23] , [24] , [25] , [26] . The schematic of the meta-device for EFISH and EFIOR is illustrated in Fig. 1a . The metamaterial absorber consists of a periodic hole array in a gold film, separated from a planar silver film by an alumina-based dielectric spacer. Each metallic layer is wired to an external circuit for voltage biasing (see Methods). Such device architecture immediately offers several features that are beneficial to the generation of EFISH and EFIOR signals. First, the nanometallic films forming the metamaterial naturally serve as electrodes for electrical input. Second, the thin dielectric gap of ~100 nm enables the generation of a giant static field within the insulating layer with modest, chip-level voltage signals. Finally, optical energy within the operational band is effectively trapped within the metamaterial absorber, thus enhancing the light concentration inside the cavity-like spacer by a factor of ~50. Similar to all nonlinear frequency-mixing processes, the efficiencies of the EFISH and EFIOR effects are positively correlated to the local intensity within the nonlinear medium, in our case, the dielectric gap. 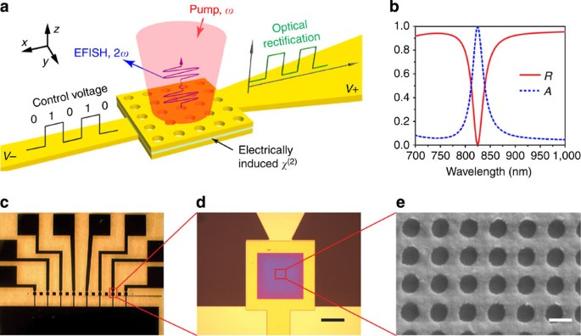Figure 1:Electrically controlled SHG and OR in a metamaterial absorber. (a) Schematic of the metamaterial device consisting of a 50-nm-thick perforated gold film, separated from an unpatterned silver layer by a 100-nm-thick alumina (Al2O3) spacer. Diameter and square lattice periodicity of the hole array are 186 and 370 nm, respectively. With connections to external circuit, the metallic layers also serve as electrodes for the voltage control. (b) Simulated reflection (R) and absorption (A) spectra indicate the perfect absorption response around the wavelength of 820 nm, whereA(ω)=1−R(ω)−T(ω) and the transmissionT(ω)=0 due to the optically thick silver layer. (c,d) Microscopic images of the entire chip with multiple EFISH devices and a close view of an individual device with electrical contacts. Scale bar, 100 μm. (e) Scanning electron microscopy image of the patterned top film of the metamaterial absorber. Scale bar, 300 nm. Figure 1: Electrically controlled SHG and OR in a metamaterial absorber . ( a ) Schematic of the metamaterial device consisting of a 50-nm-thick perforated gold film, separated from an unpatterned silver layer by a 100-nm-thick alumina (Al 2 O 3 ) spacer. Diameter and square lattice periodicity of the hole array are 186 and 370 nm, respectively. With connections to external circuit, the metallic layers also serve as electrodes for the voltage control. ( b ) Simulated reflection ( R ) and absorption ( A ) spectra indicate the perfect absorption response around the wavelength of 820 nm, where A ( ω )=1− R ( ω )− T ( ω ) and the transmission T ( ω )=0 due to the optically thick silver layer. ( c , d ) Microscopic images of the entire chip with multiple EFISH devices and a close view of an individual device with electrical contacts. Scale bar, 100 μm. ( e ) Scanning electron microscopy image of the patterned top film of the metamaterial absorber. Scale bar, 300 nm. Full size image The alumina dielectric spacer and its metallic interfaces within the metamaterial perfect absorber provide the necessary characteristics to demonstrate the EFISH and EFIOR generation. Owing to the limited magnitude of χ (3) in most materials, the realization of the EFISH or EFIOR generation typically requires a high-intensitty light source and/or a gigantic control voltage across a bulk nonlinear medium with macroscopic dimensions. These stringent requirements are substantially mitigated in the metamaterial-based platform, thanks to the deeply subwavelength thickness of the dielectric spacer and the light-concentrating ability of the metamaterial absorber. More importantly, within the absorption range of around 820 nm ( Fig. 1b ), the electric field component of the incident light is enhanced by nearly one order of magnitude, predominately perpendicular to the metal-dielectric layers and collinear with the control field. Consequently, the applied control field E c,z couples with the strongest elements in the third-order nonlinear tensor, , to create an effective second-order susceptibility in the spacer, which works together with an enhanced optical field E z ( ω ) to produce the nonlinear dipole sources for the EFISH and EFIOR fields. Linear and nonlinear spectral characteristics In this experiement, the electrically active metamaterial device is wired to an external circuit via on-chip connections, as illustrated in Fig. 1c–e . We first performed a comprehensive measurement of the nonlinear optical signals from the meta-device when excited with a tunable ultrafast laser, without an applied control voltage. Although the alumina spacer and metals used in the metamaterial are amorphous with inversion symmetry, second-order nonlinear responses are still possible, due to the symmetry breaking at the metal-dielectric interfaces [27] , [28] . 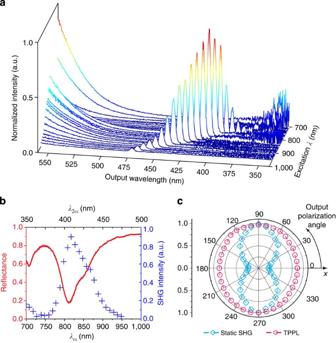Figure 2:Nonlinear optical signals from the metamaterial absorber without the application of electrical control. (a) Observed spectra of the generated nonlinear output when the metamaterial is pumped at a series of excitation wavelengths of a constant intensity. Each curve corresponds to the generated spectrum at one excitation wavelength and features a second harmonic peak atλω/2 situated on a broadband background of TPPL. (b) Measured wavelength dependence of the linear reflectance (red solid curve) and the SHG excitation spectrum (blue cross symbols), which corresponds to the peaks of the frequency-doubled output obtained ina. (c) Polarization properties of SHG (cyan squares) and TPPL (pink circles) in the absence of applied voltage. Data are normalized to their respective maximum values. The pump light is linearly polarized along the 0° direction in the polar diagram (that is, thexaxis inFig. 1a). Figure 2a shows the spectra of the produced nonlinear optical signals when the metamaterial absorber is excited at a constant intensity and the fundamental wavelength varies between 0.7−1 μm. For each pump wavelength, the output spectrum features a frequency-doubled peak at λ 2 ω = λ ω /2, which is accompanied by a broadband background of two-photon photoluminescence (TPPL) skewed towards longer wavelengths [29] . Although TPPL is known to be more efficient when pumped at relatively short wavelength, the spectral data in Fig. 2a indicates that it is enhanced, to a certain extent, by the resonance effect at the excitation wavelength of ~810 nm. Figure 2: Nonlinear optical signals from the metamaterial absorber without the application of electrical control . ( a ) Observed spectra of the generated nonlinear output when the metamaterial is pumped at a series of excitation wavelengths of a constant intensity. Each curve corresponds to the generated spectrum at one excitation wavelength and features a second harmonic peak at λ ω /2 situated on a broadband background of TPPL. ( b ) Measured wavelength dependence of the linear reflectance (red solid curve) and the SHG excitation spectrum (blue cross symbols), which corresponds to the peaks of the frequency-doubled output obtained in a . ( c ) Polarization properties of SHG (cyan squares) and TPPL (pink circles) in the absence of applied voltage. Data are normalized to their respective maximum values. The pump light is linearly polarized along the 0° direction in the polar diagram (that is, the x axis in Fig. 1a ). Full size image To elucidate the resonance behaviour of the SHG efficiency in the narrow-band metamaterial absorber, we collected the information in the frequency-doubled peaks in Fig. 2a and integrated to produce the SHG excitation spectrum shown in Fig. 2b . Also included in Fig. 2b is the measured linear reflection spectrum. As expected, the SHG reaches its peak value when pumped near the linear reflection dip because of the device’s absorption maximum at 810 nm. Similar correlations between nonlinear optical generation and linear resonance behaviour have been observed in other plasmonic systems, including textured nano-apertures and arrayed nano-antennas [30] , [31] . The slight 10 nm redshift of the SHG excitation peak relative to the linear absorption maximum is likely attributed to the damping of this resonating optical system [32] . The two components of the generated nonlinear signal are not only distinguished by the spectral features associated with SHG and TPPL but also by the distinct polarization behaviours of these two frequency up-conversion processes. As shown in Fig. 2c , the polarization of SHG emission is predominantly directed normal to that of the fundamental wave, as governed by the second-order nonlinear tensor, while the TPPL emission stems from incoherent dipoles and is therefore randomly polarized. Tuning harmonic generation with voltage signals The voltage-controlled frequency doubling in the meta-device is directly linked to the resonance-enhanced light concentration at the fundamental wavelength, with its electrical field component predominately aligned collinear with the externally applied control field. This is made evident from the simulated electric field distribution in the dielectric spacer at both the fundamental and second-harmonic wavelengths, as shown in Fig. 3a . The SHG excitation spectrum in Fig. 2b indicates the direct correlation between the SHG efficiency and the linear resonance behaviour. For this reason, all measurements of the voltage-controlled harmonic generation were fixed at a fundamental wavelength of 810 nm, which maximized the SHG output. 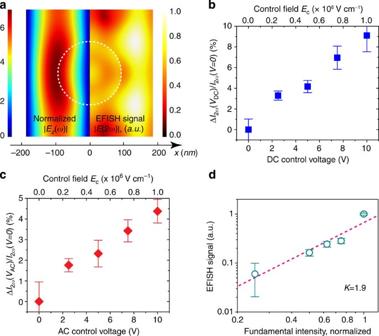Figure 3:Electrically tunable SHG in the metamaterial absorber. (a) Electric field distributions within the dielectric spacer for both the fundamental wave atω(left half, normalized to the electric field magnitude of the incident wave) and the frequency-doubled signal at 2ω(right half). The fundamental wavelength corresponds to the resonance peak where perfect absorption occurs. Only half of the unit cell is shown for each frequency because of the geometrical symmetry with respect tox=0. The white dashed circle indicates the location of the hole. (b,c) The dependence of normalized change in the frequency-doubled output ΔI2ωon the externally applied (b) DC or (c) AC voltage signals. The corresponding magnitude of the control fieldEcis labelled on the upper axis. Linearly polarized pump light at the absorption peak ofλω=810 nm was used at a fixed intensity. (d) The EFISH output ΔI2ωas a function of the intensity of the fundamental wave atλω=810 nm. The control voltage is fixed atVAC=10 V. A least-squares fit using the functionis plotted as the dashed line, in which the fit exponentKwas found to be 1.9. All error bars represent s.d. from five measurements. Figure 3b shows the change in the second-harmonic output Δ I 2 ω ( V ), normalized to the static I 2 ω ( V =0), as a function of the control field. The result reveals a linear dependence of the frequency-doubled output on the externally applied voltage, with an electric-field-induced nonlinear modulation of ~9% observed at V DC =10 V. A similar effect is obtained when the device is driven by an AC voltage signal, as shown in Fig. 3c . The linear dependence of I 2 ω on the magnitude of electrical control is beneficial for EFISH-based signal processing because electrical signals can be encoded into the frequency-doubled light generation with minimal distortion. For both the conventional SHG and the EFISH generation, the quadratic relation between SHG output and the fundamental intensity I ω is a signature characteristic. This feature is confirmed in Fig. 3d , where a slope K =1.9 of least-squares fit is identified in the double logarithmic plot. Figure 3: Electrically tunable SHG in the metamaterial absorber . ( a ) Electric field distributions within the dielectric spacer for both the fundamental wave at ω (left half, normalized to the electric field magnitude of the incident wave) and the frequency-doubled signal at 2 ω (right half). The fundamental wavelength corresponds to the resonance peak where perfect absorption occurs. Only half of the unit cell is shown for each frequency because of the geometrical symmetry with respect to x =0. The white dashed circle indicates the location of the hole. ( b , c ) The dependence of normalized change in the frequency-doubled output Δ I 2 ω on the externally applied ( b ) DC or ( c ) AC voltage signals. The corresponding magnitude of the control field E c is labelled on the upper axis. Linearly polarized pump light at the absorption peak of λ ω =810 nm was used at a fixed intensity. ( d ) The EFISH output Δ I 2 ω as a function of the intensity of the fundamental wave at λ ω =810 nm. The control voltage is fixed at V AC =10 V. A least-squares fit using the function is plotted as the dashed line, in which the fit exponent K was found to be 1.9. All error bars represent s.d. from five measurements. Full size image Electrically controlled OR In the next part of the experimental study, we characterize the OR and its electrical modulation in the metamaterial device. Under excitation of the fundamental wave, the dielectric spacer undergoes a low-frequency nonlinear polarization, causing an induced potential difference across the two metallic parts of the meta-device. The magnitude of this OR signal is critically sensitive to the level of the applied control voltage. 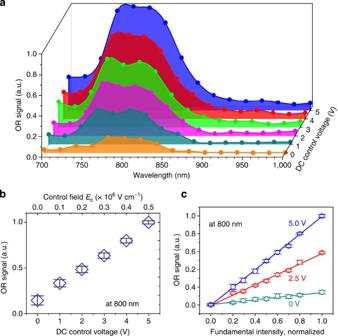Figure 4:Electrically tunable OR in the metamaterial absorber. (a) Measured excitation spectra of the OR signals under different levels of externally applied DC voltage, where the metamaterial device is excited at a series of wavelengths of constant intensity. The experimentally collected data are represented by the solid dots, and the boundaries of the coloured regions are to guide the eye. (b) The dependence of the OR output on the applied voltage when the metamaterial is pumped with fixed intensity at the wavelength of 800 nm. The corresponding magnitude of the control fieldEcis labelled on the upper axis. (c) The OR signal as a function of the intensity of the excitation light at 800 nm, when the control voltage is set to 0, 2.5 and 5 V, respectively. The solid lines are the least-squares fits to the experimental data. All error bars represent s.d. from five measurements. Figure 4a illustrates the excitation spectra of the OR signal from the metamaterial under a series of DC control voltages, from 0 to 5 V, while the excitation intensity is fixed at a constant level. All data are normalized to the peak OR signal at the bias voltage of 5 V. The experimental results reveal that the OR is strongly interrelated to the linear resonance behaviour of the metamaterial absorber. Under each control voltage, the detected rectification signal is maximized when the device is pumped at around 800 nm. This resonance characteristic near 800 nm in Fig. 4a closely follows the device’s linear absorption behaviour shown in Fig. 2b . The OR signal, which emerges as an additional, light-induced open voltage across the capacitor-like metamaterial absorber, is proportional to the corresponding quasi-DC polarization P OR ∝ I ω χ OR , where I ω is the excitation intensity and χ OR represents the effective second-order nonlinear susceptibility between the two metallic parts. The metamaterial is designed to support enhanced light intensity in the dielectric spacer within the resonance band of its linear absorption. This explains the similar resonance feature in the excitation OR spectra in Fig. 4a . Figure 4: Electrically tunable OR in the metamaterial absorber . ( a ) Measured excitation spectra of the OR signals under different levels of externally applied DC voltage, where the metamaterial device is excited at a series of wavelengths of constant intensity. The experimentally collected data are represented by the solid dots, and the boundaries of the coloured regions are to guide the eye. ( b ) The dependence of the OR output on the applied voltage when the metamaterial is pumped with fixed intensity at the wavelength of 800 nm. The corresponding magnitude of the control field E c is labelled on the upper axis. ( c ) The OR signal as a function of the intensity of the excitation light at 800 nm, when the control voltage is set to 0, 2.5 and 5 V, respectively. The solid lines are the least-squares fits to the experimental data. All error bars represent s.d. from five measurements. Full size image More importantly, the generation of OR in the metamaterial device is predominantly enabled and, therefore, can be purposely tuned by the applied control voltage. The amorphous dielectric spacer is in lack of a χ (2) response (except for the symmetry-breaking boundary), as indicated by the very limited magnitude of the OR signal in the absence of the bias voltage. The nonlinear susceptibility χ OR contributing to the OR generation is mostly electrically induced, following χ OR ∝ χ (3) E c where E c = V c / d is the applied control field. Consequently, the EFIOR signal is proportional to the bias voltage, as depicted in the inset of Fig. 4a where the magnitude of the optically rectified signal is plotted against the externally applied voltage for an excitation wavelength within the resonance band. The result indicates electrical tunability of the OR signal with a modulation depth of ~130% per volt relative to the OR level in the static ( V c =0) case. Another signature characteristic of the OR effect is the linear relation between the rectification signal and the intensity of the pump light. This is confirmed in Fig. 4b , where the OR generation is plotted as a function of the excitation intensity at the wavelength of 800 nm. At each control voltage, the slope of the least-square fit line is directly related to the electric-field-induced χ OR . To evaluate the voltage-enabled portion of rectification signal, or EFIOR, we subtract the baseline ( V c =0) from the OR data in Fig. 4b and obtain a ratio of 1.93 between the two slopes of OR curves at the control voltage of 5 and 2.5 V, respectively, which confirms the relation χ OR ∝ χ (3) E c that governs the EFIOR generation in the metamaterial absorber. We conducted a range of control measurements to confirm that no detectable SHG emission or OR beyond the noise level from the bare substrate or unpatterned metallic devices exists. This confirms that the observed nonlinear signals originate from a light concentration effect in the metamaterial absorber. As for the up-conversion efficiency of the EFISH process, we take into account all the experimental factors and conservatively estimate the efficiency to be 2 × 10 −11 . This magnitude of efficiency is comparable with the reported value for the plasmonic EFISH device [17] and that of conventional nonlinear crystals under a similar experimental condition. When both the second- and the third-order nonlinear susceptibilities are present, the total SHG intensity I 2 ω from the nonlinear medium becomes , where I ω represents the intensity of the fundamental beam and E c is the static or low-frequency electric field resulting from the control voltage. Therefore, in the EFISH generation the voltage-induced component of SHG can be expressed as . Consequently, the comparative magnitudes of χ (2) and χ (3) E c determine whether the relation Δ I 2 ω ( V c ) is quasi-linear or quasi-quadratic. The linear modulation for both DC and AC control voltage indicates that the 2 χ (3) χ (2) E c term, which depends on both χ (2) and χ (3) , dominates over the [ χ (3) E c ] 2 term in our experiment. The electrical tunability of the OR signal is much larger than that of the EFISH process, primarily because of the low level of the baseline OR in absence of an applied voltage. Without a control field, the OR-induced potential difference across the meta-device stems only from the residual χ (2) response in the gap, while in SHG the entire metallic pattern can contribute to the overall frequency-doubled output. In conclusion, we have demonstrated an electrically active nonlinear metamaterial device, in which SHG and OR can be purposely controlled by applied voltage signals. Our result leverages some of the most fascinating characteristics of optical metamaterials, namely the dual electrical and optical functionality supported by nanostructured metals, the resonance-enhanced light-matter interactions and the micrometre-scale device footprint with engineered nanoscale features. This work substantially broadens the scope of metamaterial research in the nonlinear regime and represents a key step towards using optical metamaterials as a self-sufficient platform for electro-optic information processing. Device fabrication The fabrication of the meta-device, including the external electrical wiring, involves the following procedures. First, a 100-nm-deep trench was defined by photolithography and reactive ion etching of a glass substrate. Next, the bottom electrical silver pad, which formed a flat platform for subsequent steps, was formed by depositing and lifting off a 100-nm silver layer on the predefined trench. Subsequently, aluminum oxide was deposited by both electron beam evaporation and atomic layer deposition, with a combined thickness of 100 nm. Alumina, deposited via atomic layer deposition, ensured the perfect electrical insulation and prevented electric breakdown when voltage signal was applied. On top of the aluminum oxide, aligned e-beam lithography followed by e-beam evaporation was carried out to create the upper patterned gold layer. Finally, the top electrical pad was created using another run of aligned photolithography followed by wet etching on the gold layer. The detailed fabrication procedure is described in Supplementary Fig. 1 and Supplementary Note 1 . Optical characterization The linear spectrum of the micrometre-scale device was measured using a home-made confocal system based on a tungsten–halogen lamp, a monochromator and an InGaAs detector. In the nonlinear experiments ( Supplementary Fig. 2 ), the excitation source for the experimental study was a Ti:sapphire ultrafast oscillator (Spectra-Physics, Mai Tai HP) with a pulse duration of 100 fs, a repetition rate of 80 MHz and a tuning range of 690–1,040 nm. A set of Glan polarizers and half waveplates were employed to control the power level and polarization state of excitation pulses. The fundamental beam was delivered to the metamaterial device mounted under an inverted optical microscope (Zeiss, Axio Observer D1m) with a × 10 objective, which resulted in a spot size of ~70 μm on the sample. The time-averaged power impinging on the sample was 60 mW, which translates to a peak intensity of 2 × 10 8 W cm −2 . Using a switchable beamsplitter, the generated nonlinear signals from the sample were alternatively delivered into either a photomultiplier (Hamamatsu, H10721-210) or a spectrograph system (Princeton Instruments IsoPlane and Pixis charge-coupled device camera) for intensity and spectral analysis. A dispersive prism cascaded with short-pass and band-pass filters were used to prevent the fundamental wave and the broad TPPL background from entering the photomultiplier. To test the electrical modulations of SHG with DC and AC voltage signals, lock-in measurements were performed with the input of the detector locked to either an optical chopper or a signal generator. To obtain a full spectral analysis of the nonlinear signals, the fundamental wave was filtered by a long-pass filter. This way, the broad spectrum, including both the SHG and the TPPL, was recorded using the spectrograph system. For the detection of OR, a similar lock-in setup was employed with the generated electrical signal locked to the optical chopper, in which OR signals were evaluated as a time-averaged discharging current from the capacitor-like meta-device. This current signal is proportional to the light-induced additional voltage generated across the two metallic layers, which stems from the line integral of the OR electric field across the dielectric spacer of the metamaterial. We note that the detected current signal is a direct consequence of OR, and the control voltage of a constant level does not produce this current in the absence of excitation with ultrashort laser pulses. In addition, a spectrometer at port a and a video camera on microscope at port e were used to monitor the pulse status of the Ti:sapphire oscillator and the beam alignment at the sample, respectively. All measurements were conducted under ambient temperature. Numerical simulations Full-wave numerical models of both the linear and the nonlinear properties of the metamaterial devices were performed by modifying the equation system of a commercial finite-element package (C OMSOL ). For the linear optical behaviour, the light absorption was computed as a function of the wavelength and the angle of incidence ( Supplementary Fig. 3 ). Two coupled electromagnetic models, one for the fundamental and the other for the SHG, were used in the nonlinear modelling and were solved interactively to generate the field distributions of both waves. The simulated results reveal the correlation between EFISH generation from the metamaterial absorber and the absorption behaviour of the metamaterial for the fundamental wave ( Supplementary Fig. 4 ). The intensity of the EFISH output peaks at the excitation wavelength where the linear reflectance reaches the minimum, a rather intuitive conclusion given the quadratic dependence of EFISH generation on the local intensity of the fundamental light. The nonlinear signals from the device were further evaluated using a near-to-far-field transformation technique, where the distribution and intensity of the frequency-doubled output in the far zone were calculated based on the simulated data of SHG in the close proximity of the device [33] , [34] . Specifically, all vector components of the electromagnetic fields at the harmonic frequency were obtained using unit-cell-based simulations. A virtual surface, 500 nm above the top surface of the metamaterial, was selected as the source of the far-field radiation, on which the surface electric and magnetic currents were computed from the simulated field distributions. As described by the surface equivalence theorem, the radiated fields above this virtual surface are uniquely determined by the equivalent currents on the surface. The currents’ information was further translated to vector potentials, based on which angular distribution of light in the far field can be obtained by evaluating the time-averaged Poynting vector per unit solid angle ( Supplementary Fig. 5 ). The normalized angular distribution of the EFISH power in the far field indicates relatively weak radiation near the surface normal of the metamaterial absorber. Given the × 10 objective used in our experiment with a numerical aperture of 0.25, ~8% of the entire generated EFISH signal enters the objective for further optical detection. The collection efficiency could be potentially improved by better design of the top metallic patterns such that the 2 ω signal from the metamaterial radiates with a better, controlled directionality in the EFISH process. How to cite this article: Kang, L. et al . Electrifying photonic metamaterials for tunable nonlinear optics. Nat. Commun. 5:4680 doi: 10.1038/ncomms5680 (2014).